A pH-responsive T1-T2dual-modal MRI contrast agent for cancer imaging Magnetic resonance imaging (MRI) is a non-invasive imaging technology to diagnose health conditions, showing the weakness of low sensitivity. Herein, we synthesize a contrast agent, SPIO@SiO 2 @MnO 2 , which shows decreased T 1 and T 2 contrast intensity in normal physiological conditions. In the acid environment of tumor or inflamed tissue, the manganese dioxide (MnO 2 ) layer decomposes into magnetically active Mn 2+ (T 1 -weighted), and the T 1 and T 2 signals are sequentially recovered. In addition, both constrast quenching-activation degrees of T 1 and T 2 images can be accurately regulated by the silicon dioxide (SiO 2 ) intermediate layer between superparamagnetic iron oxide (SPIO) and MnO 2 . Through the “dual-contrast enhanced subtraction” imaging processing technique, the contrast sensitivity of this MRI contrast agent is enhanced to a 12.3-time difference between diseased and normal tissue. Consequently, SPIO@SiO 2 @MnO 2 is successfully applied to trace the tiny liver metastases of approximately 0.5 mm and monitor tissue inflammation. Magnetic resonance imaging (MRI) is the most powerful technique for noninvasive tomographic imaging of biological targets for its high spatial resolution, unlimited penetration depth, and soft tissue discrimination ability [1] , [2] , [3] , [4] , [5] . However, MRI still suffers from its low inherent sensitivity, which limits the applications for diagnosis at an early stage of disease and small lesions [6] , [7] , [8] , [9] , [10] . In MRI, the relaxation time of water protons is measured, and contrast agents can alter locoregional magnetic fields and accelerate proton relaxation processes, subsequently enhancing the MRI sensitivity and diagnostic accuracy. Paramagnetic materials, which facilitate the spin-lattice relaxation of protons causing a positive MRI, are called T 1 contrast agents. T 2 contrast agents, mainly referred to as iron oxide (SPIO), cause protons in their vicinity to undergo spin-spin relaxation, which displays negative contrast on T 2 -weighted MRI images. Compared with single-mode contrast agents [11] , [12] , [13] , [14] , [15] , [16] , recently, T 1 –T 2 dual-modal MRI contrast agents can significantly improve diagnostic accuracy by providing paired anatomical images at the same levels but with different contrasts [17] , [18] , [19] , [20] , [21] , [22] . Moreover, the activatable MRI contrast agents that can recognize tumor microenvironments and change their contrasts, will also enhance the differences between normal and disease tissues [23] . Cheon and co-workers reported a magnetism-based nanoscale distance-dependent magnetic resonance tuning (MRET) system [24] . In MRET, the T 1 –weighted signal of a paramagnetic contrast agent will be quenched by a superparamagnetic T 2 contrast agent at a critical distance and recovers when they separate apart. Such MRET systems could be designed sensitively in response to biological events, such as enzymolysis, pH variation, and protein-protein interaction, realizing sensitive detection in vivo. It is no doubt that utilizing a T 1 and T 2 two-way activatable contrast agent for T 1 –T 2 dual-modal MRI will result in doubly improved detection sensitivity. In our previous work [25] , we brought the T 1 and T 2 contrast agents together in the micelles and found both the signals on T 1 and T 2 weighted MRI images were significantly reduced. When the presence of GSH disassembled the micelle structure, the MRI signals on T 1 and T 2 weighted images were dually recovered as the T 1 and T 2 contrast agents dissociated apart. Therefore, both T 1 and T 2 contrast differences were produced between the diseased and normal tissues by responding to the GSH biomarker. Further, by a method called “dual-contrast-enhanced subtraction imaging (DESI)”, the T 1 and T 2 contrast differences can be overlaid to enhance the imaging sensitivity. This work inaugurates an era for T 1 –T 2 dual-mode MRI detection. In this work, a pH-activatable T 1 –T 2 dual-modal MRI contrast agent, SPIO@SiO 2 @MnO 2 , is designed and synthesized. In the normal tissue, MnO 2 acts as an inactive T 1 contrast agent precursor, which can efficiently quench the T 2 weighted signal of SPIO. In tumor or inflammation tissue with an acid environment, MnO 2 decomposes into Mn 2+ and sequentially increases both T 1 and T 2 weighted signals. The images are further processed by the DESI method; [25] the biggest contrast difference of 12.3 times between diseased and normal tissue has been reached (Fig. 1 ). Different from the MRET with a critical distance, the quenching effect from MnO 2 to the T 2 -weighted signal of SPIO is found reversely proportional to their separation distance, i.e., the closer the quenching effect becomes stronger. As a result, both contrast quenching-activation degrees of T 1 and T 2 images can be accurately tuned by regulating the distance between SPIO and MnO 2 through the SiO 2 intermediate layer. Finally, we demonstrate that SPIO@SiO 2 @MnO 2 nanoprobe can sensitively offer high-quality image information by distance regulation and be applied to detect small lesions and identify the various acid environment. Fig. 1: Schematic illustration of the structure, working mechanism, and applications of the pH-responsive T 1 and T 2 dual-modal contrast agent. a The synthesis and structure of the contrast agent SPIO@SiO 2 @MnO 2 (SSM). SPIO represents superparamagnetic iron oxide and TEOS represents tetraethyl orthosilicate; b SPIO@SiO 2 @MnO 2 shows weak T 1 and T 2 contrast intensity in normal physiological conditions, as the T 2 signal of SPIO is quenched by the MnO 2 layer. In the acid environment of tumor or inflamed tissue, the MnO 2 layer will decompose into magnetically active Mn 2+ (T 1 -weighted), and the T 1 and T 2 signals are sequentially recovered. c Using dual-contrast-enhanced subtraction imaging (DESI) strategy enhances the imaging quality for disease diagnosis. Full size image Dual-activatable mechanism of MRI T 1 and T 2 contrast signals In this study, the nanohybrids with core/shell/shell structures were synthesized, in which the T 2 core was the superparamagnetic iron oxide (SPIO) nanoparticle. The first shell was a SiO 2 layer, and a thin layer of MnO 2 was deposited as the second shell. The final nanoparticle (SPIO@SiO 2 @MnO 2 ) was named SSM, whose core–shell-shell structure was confirmed by TEM characterization (Fig. 2a ). The size of the SPIO core was determined to be about 12.8 nm, and the thickness of SiO 2 and the MnO 2 shell were 12.4 nm and 2.2 nm. Consistently, the hydrodynamic diameter of SSM measured by DLS was 43.8 nm (Fig. 2b ). The UV–vis spectrum of SSM showed a characteristic absorption peak at 302 nm (Fig. 2c ), which could be assigned to the absorbance of MnO 2 [26] . Fig. 2: Characterization of SSM (SPIO@SiO 2 @MnO 2 ) and the pH-activatable properties. a TEM micrograph and b size distribution of SSM. Representative data are shown from three independently repeated experiments. c Absorption spectra of SS (SPIO@SiO 2 ), MnO 2 , and SSM. d T 1 Map & R 1 , and e T 2 Map & R 2 of SSM, at pH 7.4 and 5.0 respectively. T 1 and T 2 Map are representative data from three independent samples. R 1 and R 2 data are presented as mean ± SD from three independent samples. f illustration of the dual pH-activatable mechanism. g EPR spectroscopic analysis of SS at pH 7.4 and SSM at pH 7.4 and 5.0. h VSM analysis of SS at pH 7.4 and SSM at pH 7.4 and 5.0. i EDX element mapping images of SSM at pH 7.4 and 5.0 for Fe, Si, and Mn. Representative data are shown from two independently repeated experiments. Source data are provided as a Source Data file. Full size image The magnetic properties of SSM were investigated. As shown in Supplementary Fig. 1 , no resonance was observed in the electron paramagnetic resonance (EPR) spectrum of pure MnO 2 , illustrating the unpaired electrons in manganese atoms were “locked” in the oxidation state. Accordingly, SSM showed a quenched T 1 signal. According to the vibrating sample magnetometer (VSM) test in Fig. 2h , SSM showed a marked reduction in magnetization in comparison with SPIO@SiO 2 (SS), which demonstrated that MnO 2 would shield the magnetic field of the SPIO core. Therefore, in addition to the quenched T 1 weighted signal, SSM also showed a quenched T 2 weighted signal. The dual “signal quenching” property of SSM would promise a low background in imaging applications. For the quenching and activation of the T 1 signal, it is well known that the MnO 2 layer is pH -sensitive [27] , which will decompose into magnetically active Mn 2+ at the acid condition and significantly change the MRI signal of SSM. Thus, the pH sensitivity of SSM nanoparticles was investigated by measuring the MRI signals in buffers with pH values of 7.4 and 5.0, respectively. From the MRI map images in Fig. 2d, e , both T 1 and T 2 (T 1 = Longitudinal relaxation time; T 2 = Transverse relaxation time) were decreased as the pH value changed from 7.4 to 5.0. Both R 1 and R 2 values ( R 1 = 1/T 1 , R 2 = 1/T 2 ) were low at pH 7.4 and raised at pH 5.0. Thus, these results indicated that SSM showed dual-activatable T 1 and T 2 contrasts in response to the acid environment, which was believed to be the result of the decomposition of the MnO 2 outer layer. In the electron paramagnetic resonance (EPR) measurements of Fig. 2g , SSM at a pH value of 7.4 and SS showed similar doublet resonances at around 2950 and 3650 Gauss, which were the characteristic resonances of SPIO. Whereas after incubation at pH 5.0, SSM exhibited the typical peaks of Mn 2+ in addition to the peaks of SPIO. Those EPR results suggest that MnO 2 on the surface of SSM decomposed and released Mn 2+ under the acid condition, which was visibly confirmed by the EDS mapping images of SSM at pH 7.4 and 5.0 (Fig. 2i ). The decomposition of the MnO 2 shell led to two sequential results: the magnetically active Mn 2+ was released and turned on the T 1 weighted signal (the interaction between Mn 2+ and surrounding water will shorten the longitudinal relaxation times of water protons), moreover, which further eliminated the MnO 2 shield to the magnetic field of the SPIO core and resulted in “recovered” T 2 contrast signal. According to the VSM analysis (Fig. 2h ), SSM in its intrinsic state showed reduced magnetic saturation values, which corresponded to the quenched T 2 contrast signal of SSM; After being incubated at pH 5.0, SSM uncovered its MnO 2 shell, which recovered the magnetic field of the SPIO core to the original state (identified by SS). These results could well explain the pH-activatable T 2 contrast signal, which is the sequential result of the turn-on of the T 1 contrast signal. The dual activation mechanism was summarized in Fig. 2f , which determined that SSM would show high sensitivity in discriminating the diseased (with the acid environment) and normal tissues (with the neutral environment). The mechanism of the quenching effect on T 2 contrast signal According to the above investigations on the SSM contrast agent, we observed that the T 1 contrast signal of Mn 2+ was “masked” by the formation of MnO 2 . Moreover, the MnO 2 would quench the T 2 contrast signal of the SPIO subsequently, resulting in the “dually (T 1 and T 2 ) quenched” state of the contrast agent in the neutral condition. Like one key for two locks, the decomposition of MnO 2 could efficiently convert the contrast agent into the “dually (T 1 and T 2 ) activated” state in the acid environment. It has been clearly proved that the T 1 contrast signal of a T 1 contrast agent (paramagnetic properties) will be quenched by a T 2 contrast agent (superparamagnetic properties) when their distance becomes close enough [24] . Therefore, we further tuned the distance between the SPIO core and the MnO 2 layer by varying the thickness of the intermediate SiO 2 layer. The thickness of the silica shell can be adjusted by controlling the reaction time (Supplementary Fig. 2 ). 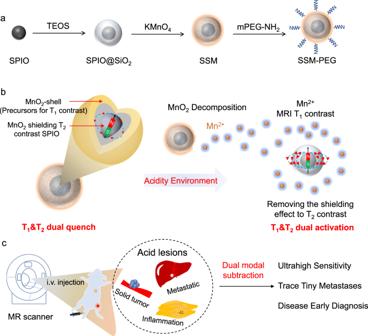Fig. 1: Schematic illustration of the structure, working mechanism, and applications of the pH-responsive T1and T2dual-modal contrast agent. aThe synthesis and structure of the contrast agent SPIO@SiO2@MnO2(SSM). SPIO represents superparamagnetic iron oxide and TEOS represents tetraethyl orthosilicate;bSPIO@SiO2@MnO2shows weak T1and T2contrast intensity in normal physiological conditions, as the T2signal of SPIO is quenched by the MnO2layer. In the acid environment of tumor or inflamed tissue, the MnO2layer will decompose into magnetically active Mn2+(T1-weighted), and the T1and T2signals are sequentially recovered.cUsing dual-contrast-enhanced subtraction imaging (DESI) strategy enhances the imaging quality for disease diagnosis. As a consequence, different SSM nanoparticles were synthesized with different SiO 2 thicknesses (4, 8, and 12 nm) but the same amounts of SPIO and MnO 2 , which had been verified via ICP-MS analysis (Supplementary Table 1 ). 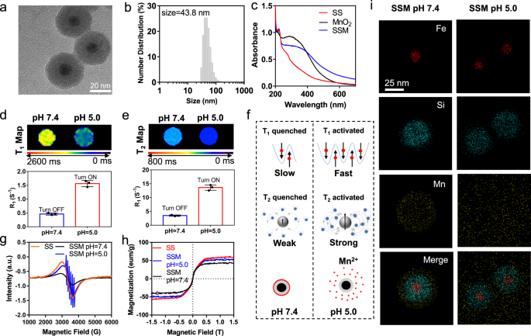Fig. 2: Characterization of SSM (SPIO@SiO2@MnO2) and the pH-activatable properties. aTEM micrograph andbsize distribution of SSM. Representative data are shown from three independently repeated experiments.cAbsorption spectra of SS (SPIO@SiO2), MnO2, and SSM.dT1Map & R1, andeT2Map & R2of SSM, at pH 7.4 and 5.0 respectively. T1and T2Map are representative data from three independent samples. R1and R2data are presented as mean ± SD from three independent samples.fillustration of the dual pH-activatable mechanism.gEPR spectroscopic analysis of SS at pH 7.4 and SSM at pH 7.4 and 5.0.hVSM analysis of SS at pH 7.4 and SSM at pH 7.4 and 5.0.iEDX element mapping images of SSM at pH 7.4 and 5.0 for Fe, Si, and Mn. Representative data are shown from two independently repeated experiments. Source data are provided as a Source Data file. 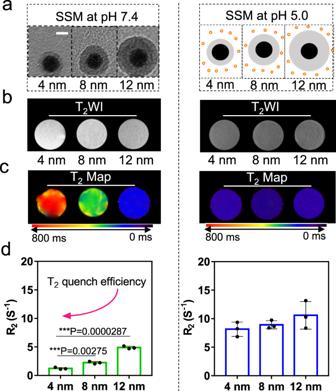Fig. 3: The distance-dependent quenching effect of MnO2to T2contrast signal of the SPIO core. aTEM images and schematic illustration of the structure of SSM (SPIO@SiO2@MnO2) with different SiO2thicknesses (4, 8, and 12 nm) at pH 7.4 and 5.0, scale bar = 12 nm. The SiO2intermediate layer works as a ruler to investigate the influence of distance on the T2quenching effect;bT2-weighted images,cT2Map, anddR2of SSM samples with different SiO2thicknesses (4, 8, and 12 nm) at pH 7.4 and 5.0. T2-weighted images and T2Map are representative data from three independent samples.R2data are presented as mean ± SD from three independent samples. The two-tailed Student’st-test is employed for the statistical analysis. *P< 0.05; **P< 0.01; ***P< 0.001. Source data are provided as a Source Data file. Figure 3a presents the TEM image of these SSM nanoparticles and the schematic illustration of the decomposition of the MnO 2 layer in the acid environment. We evaluated the MRI performance of the three SSM nanoparticles in the neutral or acid environment. As seen from Supplementary Fig. 3 , without the coating of the MnO 2 layer, SS with different SiO 2 thicknesses showed identical R 1 values. The R 2 value of SS nanoparticles was reduced in comparison with naked SPIO. However, the R 2 values of SS nanoparticles with various thicknesses of the SiO 2 layer (4, 8, and 12 nm) showed similar intensity. The results revealed that the SiO 2 layer mainly influenced the surface properties. After coating the MnO 2 layer, the T 1 signal showed no significant change with the SiO 2 thickness decreasing (Supplementary Fig. 4 ), which was reasonable as MnO 2 showed no magnetic activity. While the T 2 weighted images of SSM dramatically changed from dark gray to bright (Fig. 3b ), and the T 2 signal was significantly decreased with decreasing the SiO 2 thickness, as observed from the Map image in Fig. 3c and R 2 value in Fig. 3d . All these results proved that the MnO 2 layer would shield the magnetic field of the SPIO core, and the shielding effect became more significant as the MnO 2 layer approached the SPIO core. Fig. 3: The distance-dependent quenching effect of MnO 2 to T 2 contrast signal of the SPIO core. a TEM images and schematic illustration of the structure of SSM (SPIO@SiO 2 @MnO 2 ) with different SiO 2 thicknesses (4, 8, and 12 nm) at pH 7.4 and 5.0, scale bar = 12 nm. The SiO 2 intermediate layer works as a ruler to investigate the influence of distance on the T 2 quenching effect; b T 2 -weighted images, c T 2 Map, and d R 2 of SSM samples with different SiO 2 thicknesses (4, 8, and 12 nm) at pH 7.4 and 5.0. T 2 -weighted images and T 2 Map are representative data from three independent samples. R 2 data are presented as mean ± SD from three independent samples. The two-tailed Student’s t -test is employed for the statistical analysis. * P < 0.05; ** P < 0.01; *** P < 0.001. Source data are provided as a Source Data file. Full size image To reveal the mechanism of T 2 signal quenching, we analyzed the T 2 weighted signal of the SPIO with different diamagnetic shells. We found that at the same SiO 2 shell thickness (4 nm), SS nanoparticles showed mild T 2 signal quenching. When further coating Ag 2 O and MnO 2 , the nanoparticles showed enhanced T 2 signal quenching (Supplementary Fig. 5 ). Therefore, the diamagnetic nature of the MnO 2 or Ag 2 O layer would shield the magnetic field of the SPIO core and quench the T 2 -weighted signal to a certain degree. Similar phenomena have also been reported in other research works [28] , [29] , [30] . However, we also observed that the MnO 2 layer shows a more significant quenching effect compared with Ag 2 O and SiO 2 . For the Ag 2 O diamagnetic shell, as the distance between SPIO and Ag 2 O increased, almost no distance effect could be observed (Supplementary Fig. 6 ), which was quite different from the result of the MnO 2 diamagnetic shell. Moreover, in addition to the distance effect, we further measured the T 2 weighted image of SPIO@SiO 2 @MnO 2 at the same SiO 2 -shell thickness while changing MnO 2 contents (Supplementary Fig. 7 ). The result indicated the T 2 quenching effect was notably enhanced by changing Fe/Mn weight ratios from 1:1 to 1:40 while controlling the same SPIO amount and SiO 2 thickness. The difference between MnO 2 and Ag 2 O demonstrated that additional reasons (rather than the shielding effect of the diamagnetic shell) caused the MnO 2 layer to quench the T 2 signal of SPIO. We assumed the T 2 quenching effect also came from the negative exchange interaction between Mn and Fe, which results in a non-collinear antiferromagnetic configuration in their combination [31] . Such exchange interactions were also observed in bi-magnetic core/shell nanoparticles, which would generate a large exchange bias as the two magnetic materials were coupled together. Moreover, it was reported that such magnetic exchange interaction did show distance dependence [32] . We observed that, with a SiO 2 interlayer of 4 nm, the R 2 value of SSM showed a ~12.0 times decrease in comparison with SS (Supplementary Fig. 3 ); as a result, the T 2 contrast signal of SSM was almost completely quenched. In comparison, SSM and SS showed a 6.6-time difference for 8 nm SiO 2 interlayer and a 3.0-time difference for 12 nm SiO 2 interlayer in R 2 values (Fig. 3d left). After the decomposition of the MnO 2 shell in an acid environment (pH=5.0), the R 2 values of all three nanoparticles recovered to the same level (Fig. 3d right). At pH 7.4, the transverse relaxivity r 2 of SSM with various SiO 2 thicknesses of 4, 8, and 12 nm were 12.08, 21.06, and 35.38 mM −1 s −1 , respectively. On the contrary, r 2 values of SSM at pH 5.0 showed no notable differences (Supplementary Fig. 8 ). These results suggested that the shielding effect of the MnO 2 layer on the SPIO core was distance-dependent. Therefore, the contrast sensitivity of the SSM probe can be accurately tuned by regulating the thickness of the SiO 2 intermediate layer. The SSM nanoparticle with a 4 nm SiO 2 layer was used for all the following experiments. The longitudinal relaxivity ( r 1 , 1.34 and 4.60 mM −1 s −1 ) and transverse relaxivity (r 2 , 13.88 and 82.21 mM −1 s −1 ) of SSM at pH value of 7.4 and 5.0 were displayed in Supplementary Fig. 9 , the r 1 and r 2 of SSM both enhanced due to the environment pH changed from 7.4 to 5.0. MRI discriminates between the normal and cancer cells The pH-dependent MRI property of SSM nanoparticles was further investigated. As shown in Supplementary Fig. 10 , in the pH range from 7.4 to 4.0, the T 1 weighted images showed gradually “activated” signals (becoming brighter and brighter); meanwhile, the T 2 weighted images were also “activated” (becoming darker and darker). Calculated from the MRI map images in Fig. 4a , both R 1 and R 2 values were decreased as the pH value decreased. For the excellent sensitivity of SSM in pH detection, it is worth noting that there was a good linear relationship between the R 1 / R 2 values and the pH values (Fig. 4b, c ). Also, in addition to the pH-dependent properties, both the T 1 weighted image, T 1 map image, T 2 weighted image, and T 2 map image of SSM showed a time-dependent response to the acid environment (Supplementary Fig. 11 ). As SSM could sensitively indicate the change of less than 1.0 pH unit, we tried to utilize SSM as the MRI probe to discriminate between the normal and cancer cells. Generally, cancer cells showed higher glycolytic activity than normal cells; therefore, cancer cells would uptake and produce more lactate acid, resulting in acidic intracellular and extracellular environments [33] . According to the previous investigations, the pH measured at the surface of the highly metastatic cells was pH 6.7–6.8, and within tumors was around pH 6.1–6.4 [34] . As a result, metastatic cells can be 0.6–1.3 pH units lower than normal cells (pH 7.4). Three different cell lines, 293T, 4T1, and U87, were selected and incubated with SSM for 4 h. 293T is a normal cell line, while both 4T1 and U87 are highly metastatic cancer cells. From the data in Fig. 4d–f and Supplementary Fig. 12 , both the T 1 and T 2 images in the 293 T group were kept low contrast signals; on the contrary, the corresponding images in the two tumor cell groups (4T1 and U87) were all activated to high signal levels. The time dependency of dual-active MRI signals incubated in 4T1 cells and 293T cells were also investigated. As shown in Supplementary Figs. 13 , 14 and Fig. 4g, h , both the R 1 and R 2 values of the 4T1 cell group exhibited a time-dependent increasing process, whereas the 293T cell group did not show obvious changes in R 1 and R 2 values. As the cancer cells showed a more acidic intracellular environment, SSM nanoparticles showed gradually activated signals on T 1 and T 2 images along with the intracellular uptake of the SSM nanoparticles. These results proved that SSM was an MRI probe that can sensitively respond to pH changes, showing great potential in tumor and inflammation diagnosis in vivo. Fig. 4: Capability of SSM (SPIO@SiO 2 @MnO 2 ) in pH discrimination between normal and cancer cells. a T 1 Map and T 2 Map of SSM in different pH environments (pH = 7.4, 6.0, 5.0, and 4.0). Representative data are shown from three independent samples. b R 1 and c R 2 of SSM in different pH environments (pH = 7.4, 6.0, 5.0, and 4.0). Data are presented as mean ± SD from three independent samples. d T 1 Map and T 2 Map of different cell lines (293T, 4T1, and U87) incubated with SSM. Representative data are shown from three independent samples. e R 1 and f R 2 of different cell lines (293T, 4T1, and U87) incubated with SSM. Data are presented as mean ± SD from three independent samples. g R 1 and h R 2 of 293T and 4T1 cell lines incubated with SSM for different periods (0.5, 1, 2, 4, 8, and 16 h). Data are presented as mean ± SD from three independent samples. The two-tailed Student’s t -test is employed for the statistical analysis. * P < 0.05; ** P < 0.01; *** P < 0.001. Source data are provided as a Source Data file. Full size image MRI detection on the in vivo xenograft model For in vivo application, PEG 5K -NH 2 modified SSM (SSM-PEG) was synthesized to enhance the biostability and biocompatibility of the MRI probe. The PEG attached to the SSM surface was due to the Mn-N coordinate bonding between PEG-NH 2 and MnO 2 . The size and zeta potential results (Supplementary Figs. 15 and 16 ) displayed that SSM-PEG showed a larger size and more neutral surface potential in comparison with SSM due to the surface modification of PEG. Further, the T 1 and T 2 map images of SSM and SSM-PEG in different pH buffers (pH=7.4, 6.0, and 5.0) were tested and compared. The calculated R 1 and R 2 values were summarized in Supplementary Fig. 17 , demonstrating that the PEGylation modification would not affect the pH-activation process. In SSM-PEG, the SSM part could still be freely accessible to the environment as the PEG shell was hydrophilic and loosely packed. The stability test in Supplementary Fig. 18 indicated that SSM-PEG could keep stable for nearly 48 h in a 10% Fetal Bovine Serum (FBS) solution. It should be noted that the DLS analysis was conducted by the “intensity weighted distribution” method here to eliminate the interferences from a large number of FBS molecules. However, the “intensity weighted distribution” method will be more biased to the larger nanoparticles than the previously used “number weighted distribution” method; therefore, a relatively larger size of SSM-PEG was displayed. In addition, cytotoxicity tests were carried out to evaluate the safety of SSM-PEG. Both SSM and SSM-PEG exhibited no significant cytotoxicity in the 4T1 cell line after 24 h incubation (Supplementary Fig. 19 ). Moreover, the cytotoxicity of Mn 2+ was investigated (Supplementary Fig. 20 ). Mn 2+ with a concentration up to 1000 μM still showed negligible cytotoxicity (>85% viability). Therefore, considering the dosages we used, no obvious toxicity would be induced by Mn 2+ release from the SSM nanoprobe. What’s more, the Prussian blue staining experiment in Supplementary Fig. 21 proved that SSM-PEG showed a good cell uptake property. The hemolysis assay is a universal method to evaluate the hemocompatibility of materials. Thus, hemolysis study was carried out to further assess the biocompatibility of SSM-PEG. The results (Supplementary Fig. 22 ) proved that SSM-PEG displayed a low cytotoxic response at two different concentrations of 50 μg/mL and 100 μg/mL (<5% of hemolysis); on the contrary, SSM without PEGylation under the same concentrations showed marked hemolysis (>50% of hemolysis). The results demonstrated that the PEGylation was important for improving the biocompatibility of the SSM probe, making it safe for intravenous administration. The pharmacokinetics studies on SSM-PEG and SSM further proved the critical role of PEGylation in in vivo application. The blood circulation time t 1/2 of SSM-PEG increased to nearly 82.8 min (Supplementary Fig. 23 ), while t 1/2 of SSM was 29.0 min. The PEG stealth layer will protect the particle from uptake by the reticuloendothelial system and elongate the blood circulation time. Based on the good biostability and biosafety of SSM-PEG, we further investigated the feasibility of SSM-PEG as the MRI contrast agent in vivo. First, SPIO-PEG and MnO 2 -PEG were prepared as control materials to test whether SSM-PEG would well go through pH-activation in vivo in the tumor acidic environment. SPIO-PEG was synthesized in the absence of the MnO 2 layer, and MnO 2 -PEG was synthesized without the SPIO@SiO 2 core. SSM-PEG, MnO 2 -PEG (the control group of pH-activatable T 1 contrast image), and SPIO-PEG (the control group of T 2 contrast image after activation) were intravenously (I.V.) injected into the 4T1 breast subcutaneous tumor model and performed the MRI measurement. After injection, the tumor sites of the mice treated with SSM-PEG showed gradually enhanced both T 1 and T 2 contrast in the MR images, along with a time increase (Supplementary Fig. 24 ). While the mice treated with MnO 2 -PEG (Supplementary Fig. 25 ) only showed enhanced T 1 contrast in tumor image, and SPIO-PEG (Supplementary Fig. 26 ) only showed enhanced T 2 contrast. As shown in Fig. 5a–c , The T 1 contrast signals at the tumor sites were all similar for the MnO 2 -PEG and SSM-PEG groups at different time points post-injection. In contrast, SSM-PEG displayed a visibly lower T 2 contrast in comparison with SPIO-PEG at the first hour; after that, SSM-PEG and SPIO-PEG reached a similar level of MRI T 2 contrast signal at 12 h post injection. Such a phenomenon accorded with the fact that SSM-PEG needed to go through the activation process to give the MRI signals. At 12 h after injection, both the T 1 and T 2 contrast signal of the SSM-PEG group in the tumor site approached the levels same as that of SSM-PEG and SPIO-PEG, respectively, indicating the full activation of the SSM-PEG probe. Due to the T 1 &T 2 dual-modal properties of SSM-PEG after the activation in the acid-tumor environment, we could further use the dual-contrast-enhanced subtraction imaging (DESI) method to sum up the dual contrast and subsequently improve the diagnosis resolution. As shown in Fig. 5d , the DESI was carried out by subtracting the T2-weighted image from the T 1 weighted image and further inverting the resultant image. As shown in Fig. 5e–g (The details of the subtraction process and origin images were displayed in Supplementary Fig. 27 ), compared with MnO 2 -PEG and SPIO-PEG that are single-modal (T 1 or T 2 ) contrast agents, the dual-modal activatable SSM-PEG showed a significantly enhanced imaging sensitivity after the DESI treatment, the tumor site displayed remarkable dark gray MRI signal while the normal tissue showed nearly “zero” background in the SSM-PEG group. Further, the tumor-to-normal tissue signal ratios (TNRs) of the three contrast agents were quantified from their T 1 -weighted images, T 2 -weighted images, and DESI-processed images. We observed that SSM-PEG showed a similar T 1 weighted TNR and a relatively higher T 2 weighted TNR in comparison with MnO 2 -PEG; meanwhile, SSM-PEG showed a similar T 2 weighted TNR and a relatively higher T 1 weighted TNR in comparison with SPIO-PEG. Therefore, as SSM-PEG could improve both the T1-weighted TNR and the T2-weighted TNR, the DESI processing method can significantly improve the TNR value of the SSM-PEG group. In contrast, DESI processing showed no visible enhancing effect on the TNR value of the SPIO-PEG (in comparison with its T 2 weighted TNR) and MnO 2 -PEG groups (in comparison with its T 1 weighted TNR). From Fig. 5h , the TNR value for SSM-PEG quantified from the DESI processed images was 12.3 times; on the contrary, the TNR values for MnO 2 -PEG and SPIO-PEG were 3.8 and 2.1, respectively. Thus, we demonstrated that by using the T 1 &T 2 dual-activatable SSM probe and processing the MRI images through the DESI method, the resolution of in vivo MRI images could be remarkably improved. Furthermore, the Prussian blue stain (to indicate the ferric iron) in Fig. 5i and the tumor tissue TEM image in Fig. 5j, k confirmed that the SSM-PEG accumulated in the tumor site. The in vivo biocompatibility of SSM-PEG was also monitored via the blood routine examination, main organ pathological examination, and bio-distribution in vivo (Supplementary Figs. 28–30 ); all the results indicated that SSM-PEG has good biosafety in vivo. Thus, according to the MRI results on the xenograft model, it was proved that SSM-PEG could visualize the tumor site in vivo well. Fig. 5: SSM-PEG (PEG-modified SPIO@SiO 2 @MnO 2 ) for in vivo MRI of 4T1 xenograft tumor-bearing mice. a T 1 and T 2 Map, b R 1 , and c R 2 at the tumor site of the 4T1-bearing mice. The I.V. injections of SSM-PEG and MnO 2 -PEG were given a dosage of 5 mg/kg, and the MRI diagnosis was performed at different time points at 0, 1, 6, and 12 h post the injection. T 1 and T 2 Map are representative data from three mice samples. R 1 and R 2 Data are presented as mean ± SD from three independent mice samples. d Illustration of the Dual-contrast-Enhanced Subtraction Imaging (DESI) procedures; T 1 and T 2 dual-modal MRI images were processed by DESI method of the tumor-bearing mice at 12 h after the injection of e SSM-PEG, f MnO 2 -PEG, and g SPIO-PEG. Representative data are shown from three mice samples. h The tumor-to-normal tissue signal ratios (TNRs) quantified from the DESI processed images in e – g . Data are presented as mean ± SD from three independent mice samples. i Prussian blue stain and ( j ) and ( k ) TEM images of the tumor slices from the mice receiving the injection of SSM-PEG. Representative data are shown from three mice samples. The two-tailed Student’s t-test is employed for the statistical analysis. * P < 0.05; ** P < 0.01; *** P < 0.001. Source data are provided as a Source Data file. Full size image MRI detection for the metastatic model Considering that SSM-PEG can bring significant MRI contrast between the tumor and normal tissue, we attempted to use it to trace the tiny liver metastases. The metastatic model was established by splenic injection of 4T1 breast cancer cells (Fig. 6a ). By MRI monitoring, we found that liver micro-metastatic tumors were well-formed in most of the mice as early as 1 week post-injection (Supplementary Fig. 31 ). However, some of the micro-metastatic tumors had grown big in size. In one case, after the intravenous injection of SSM-PEG, a micro-metastasis (diameter less than 0.5 mm) was visible by both the T 1 -weighted and T 2 -weighted images, which could be more clearly discriminated after DESI treatment. However, without the injection of SSM-PEG, the same micro-metastasis could not be observed even using the DESI treatment (Fig. 6d ). By using the SSM-PEG contrast agent, both the signals on T 1 and T 2 map images at the liver metastasis were significantly enhanced in comparison with the normal liver tissue (Supplementary Fig. 32 and Fig. 6b–d ), while there was almost no contrast difference between the normal and tumor tissues without the injection of the SSM-PEG. The signal ratio from tumor-to-normal liver tissue (TNR) of SSM-PEG was 4.7 times via the DESI method (Fig. 6g ). Ex vivo microscopies and the H&E staining image of liver tissues in Fig. 6e, f confirmed the presence of metastatic lesions of approximately 0.5 mm. This experiment proved that the high sensitivity of the SSM-PEG contrast agent made the recognition of metastatic foci in the liver possible. Fig. 6: SSM-PEG (PEG-modified SPIO@SiO 2 @MnO 2 ) for MRI trace of tiny liver metastases in vivo. a Illustration of the construction and MRI diagnosis processes of the metastatic model. b T 1 and T 2 map images and c R 1 and R 2 at the liver metastasis of the mice before I.V. injection and 2 h after the injection of SSM-PEG. T 1 and T 2 Map are representative data from three mice samples. R 1 and R 2 Data are presented as mean ± SD from three independent mice samples. d T 1 and T 2 dual-modal MRI images of the liver metastasis were processed by DESI method, which were taken without the use of contrast agent and 2 h after the injection of SSM-PEG. Representative data are shown from three mice samples. e Ex vivo image of the liver with a tiny metastasis. Representative data are shown from three mice samples. f H&E stain of the slices of the liver metastasis. Representative data are shown from three mice samples. g TNR quantified from the DESI processed images in d and e. Data are presented as mean ± SD from three independent mice samples. The two-tailed Student’s t -test is employed for the statistical analysis. * P < 0.05; ** P < 0.01; *** P < 0.001. Source data are provided as a Source Data file. Full size image MRI detection for inflammation In the inflammation tissue, anaerobic glycolysis, lactic acid accumulation, hypoxia, and hypochlorous acid production by activated neutrophils contribute to local acidosis, also leading to an acidic microenvironment [35] , [36] . So, the pH value of the microenvironment was strongly associated with inflammation severity. On the other hand, numerous reports have revealed that nanoparticles could also accumulate in the inflammation site [37] , [38] . Therefore, we propose that dual-activatable contrast agent SSM-PEG could also be used for inflammation diagnosis. The muscle inflammation model was established by injecting turpentine into the thigh muscle of rats. After the inflammation model was established, SSM-PEG was intravenously injected for MRI detection. As shown in Fig. 7a–d , SSM-PEG through the I. V. injection could accumulate and present higher signals on T 1 and T 2 weighted and map images in the inflammation tissue in comparison with that of the normal tissue. Conversely, the inflammation foci could not be clearly observed by both the T 1 -weighted and T 2 -weighted images before the injection of SSM-PEG. The R 1 and R 2 values at the muscle inflammation sites before and after the injection of SSM-PEG contrast agents were summarized in Fig. 7e, f . Significant MRI signal changes were revealed. The H&E stain slice confirmed the presence of inflammation in muscle tissue (Fig. 7g ). All these results proved that SSM-PEG also has the potential to monitor tissue inflammation. Fig. 7: SSM-PEG (PEG-modified SPIO@SiO 2 @MnO 2 ) for MRI diagnosis of inflammation in vivo. a T 1 and T 2 weighted images and b T 1 & T 2 Map of muscle inflammation without the use of contrast agents. Representative data are shown from three mice samples. c T 1 and T 2 weighted images and d T 1 and T 2 Map of muscle inflammation of the rats receiving I.V. injection of SSM-PEG. Representative data are shown from three mice samples. e R 2 and f R 1 at the muscle inflammation sites before and after 2 h injection of SSM-PEG contrast agents. Data are presented as mean ± SD from three independent mice samples. g H&E stain of tissue slices taken from the muscle inflammation sites. Representative data are shown from three mice samples. The two-tailed Student’s t -test is employed for the statistical analysis. * P < 0.05; ** P < 0.01; *** P < 0.001. Source data are provided as a Source Data file. Full size image In summary, to improve the diagnostic sensitivity of the MRI technique, we developed an MRI contrast agent, SSM, with a core/shell/shell structure and showing T 1 and T 2 dual-activatable signals. In this structure, the MnO 2 layer is pH-sensitive, which plays a crucial role in the signal transductions from normal tissue to diseased tissue. In the normal physiological condition, we revealed that the MnO 2 shell would shield the magnetic field of the SPIO core and consequently reduce the T 2 signal. Moreover, the diminishing effect of the MnO 2 layer on the T 2 signal of the SPIO core was highly dependent on the thickness of the intermediate SiO 2 layer. The maximal decrease (~12 times) in T 2 relaxation rates could be reached if the thickness of SiO 2 was reduced to 4 nm. Based on the excellent MRI sensitivity, SSM was successfully applied to trace the tiny liver metastases of approximately 0.5 mm and to accurately monitor tissue inflammation. Overall, this research provides a design idea for a contrast agent that can provide high sensitivity for lesion detection, which shows great clinical significance in early diagnosis, prognosis, prediction, and monitoring of the recurrence of diseases. Materials Chemicals and solvents were used as received without further purification unless specified otherwise. Iron chloride, sodium oleate, oleic acid, Igepal CO-520, tetraethyl orthosilicate (TEOS), and 1-octadecene (ODE) were obtained from Aladdin Reagent (Shanghai) Co., Ltd Potassium permanganate (KMnO 4 ) and Manganese sulfate (MnSO 4 ) were purchased from Sinopharm Chemical Reagent Co., Ltd mPEG 5K -NH 2 and RhB-PEG 5K -NH 2 were obtained from Shanghai Ponsure Biotech, Inc. Other commonly used solvents were obtained from Aladdin Reagent (Shanghai) Co., Ltd. Prussian blue iron stain kit was obtained from Sangon Biotech (Shanghai) Co., Ltd. The Cell lines 4T1 (catalog number SCSP-5056), 293T (catalog number SCSP-502), and U87(catalog number TCHu138) were purchased from Cell Bank of Chinese Academy of Sciences. Cell culture materials, such as RPMI 1640 medium, DMEM, fetal bovine serum (FBS), and streptomycin/penicillin solution, were supplied by Gibco BRL Co., Ltd (Grand Island, NY, USA). 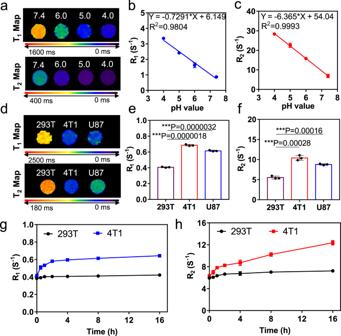Fig. 4: Capability of SSM (SPIO@SiO2@MnO2) in pH discrimination between normal and cancer cells. aT1Map and T2Map of SSM in different pH environments (pH = 7.4, 6.0, 5.0, and 4.0). Representative data are shown from three independent samples.bR1andcR2of SSM in different pH environments (pH = 7.4, 6.0, 5.0, and 4.0). Data are presented as mean ± SD from three independent samples.dT1Map and T2Map of different cell lines (293T, 4T1, and U87) incubated with SSM. Representative data are shown from three independent samples.eR1andfR2of different cell lines (293T, 4T1, and U87) incubated with SSM. Data are presented as mean ± SD from three independent samples.gR1andhR2of 293T and 4T1 cell lines incubated with SSM for different periods (0.5, 1, 2, 4, 8, and 16 h). Data are presented as mean ± SD from three independent samples. The two-tailed Student’st-test is employed for the statistical analysis. *P< 0.05; **P< 0.01; ***P< 0.001. Source data are provided as a Source Data file. BALB/c mice, nude mice and nude rats were purchased from Vital River Laboratory Animal Technology Co., Ltd (Beijing, China). Housing: ambient temperature 20–26 °C, relative humidity 40–70%, dark/light cycle 19:00–07:00/07:00–19:00. Characterizations TEM (FEI Talos F200x) was employed to observe the morphology of SPIO, SPIO@SiO 2 , and SPIO@SiO 2 @MnO 2 . The samples (1 mg mL −1 ) were made by directly dripping the nanoparticle solution onto copper grids and placed at room temperature to dry naturally. The element mapping was performed by the EDS attachment of HR TEM. Size distribution of the above nanoparticle solutions (1 mg mL −1 ) were observed by dynamic light scattering (DLS) instruments (Malvern, Nano-ZS). UV–vis absorption spectra were recorded with a Lambda 35 spectrometer (PerkinElmer, America) between 200–800 nm at 2 nm intervals. The Electron Paramagnetic Resonance (EPR) curves were recorded on a Bruker EMXplus-10/12 EPR Spectrometer. All continuous-wave EPR data were acquired under non-saturating conditions at room temperature, with an excitation microwave frequency of 9.87 GHz, microwave power of 0.6325 mW and modulation frequency of 100 kHz. Hysteresis loops were measured at room temperature using a vibrating sample magnetometer LakeShore7404. Before the test, we prepared the sample SS and SSM with the same SPIO concentration. During the test, the same volume of each type of sample was loaded into the same liquid sample holder with a cap from Lake Shore Cryotronics and filled to capacity before the measurement. Synthesis of superparamagnetic iron oxide (SPIO) SPIO was prepared through the thermal decomposition of iron-oleic acid complexes at a high temperature. In a typical synthesis, iron chloride (6.5 g, 40 mmol) was first dissolved in a mixture of 80 mL ethanol and 60 mL ultrapure water in a three-neck flask (500 mL). Afterward, sodium oleate (36.5 g, 120 mmol) was added to the iron chloride solution along with 140 mL hexane. After the complete dissolution, the reaction solution was heated to ~ 70 °C for 4-h reflux, then the upper organic layer containing the iron oleate was washed three times with ultrapure water and placed under a vacuum at 60 °C overnight. Iron oleate (3 mmol, 2.7 g) and oleic acid (1.65 mmol, 0.468 g) were added into a three-neck flask with 15 g ODE as solvent. The mixture was stirred under Argon flow at 100 °C. After 30 min, the mixture was heated to 300 °C at a rate of 18 °C/min. After 1 h, the reaction solution was quickly cooled, and the resulting products were precipitated by acetone, then purified three rounds by acetone/hexane. The final product was dispersed in cyclohexane. Synthesis of SPIO@SiO 2 A reverse microemulsion method was used to prepare SPIO@SiO 2 core−shell nanoparticles. Typically, 0.25 g Igepal CO-520 was dispersed in 5 mL of cyclohexane, and the resultant solution was sonicated for 5 min. Then, the solution of 12-nm SPIO (10 mg mL −1 , 100 μL) was added to the above solution and sonicated for 5 min. Subsequently, 50 μL of ammonium hydroxide was added and sonicated for another 5 min. Finally, TEOS (2 μL) was added, and the mixture was placed in a flip shaker. The reaction time was set as 2, 6, and 16 h to control the shell thickness of SiO 2 . Finally, 2 mL ethanol was added to stop the reaction, and the products were centrifuged and washed three times by ethanol and ultrapure water, respectively. The obtained SPIO@SiO 2 was finally dispersed in 1 mL ultrapure water for use. Synthesis of SPIO@SiO 2 @MnO 2 (SSM) As prepared SPIO@SiO 2 (1 mL) was mixed with the KMnO 4 solution (1 mg mL −1 in water, 1.58 mL), and the mixture was stirred for 5 min. Then, the MnSO 4 solution (1 mg mL −1 , 2.26 mL) was added dropwise into the above mixture. After 4 h, the products were collected by centrifugation and then washed by water three times. Finally, the product was placed on the magnetic separation rack overnight, and then the separated SPIO@SiO 2 @MnO 2 product was dissolved in 1 mL ultrapure water for future use. For the T 1 control group, MnO 2 was prepared using the same method just without the addition of SPIO@SiO 2 at the very beginning. Synthesis of SPIO@SiO 2 @MnO 2 -PEG (SSM-PEG) To prepare SPIO@SiO 2 @MnO 2 -PEG, 2 mg of mPEG-NH 2 was added to a solution of SPIO@SiO 2 @MnO 2 (1 mg mL −1 , 1 mL), and then the mixture was placed in a flip shaker for 24 h. The resulting SPIO@SiO 2 @MnO 2 -PEG product was purified by magnetic separation to remove the unreacted mPEG-NH 2 . The biocompatible T 1 control group MnO 2 -PEG was prepared using the same method by the addition of MnO 2 at the very beginning. MRI performance The T 1 -weighted imaging (T 1 WI), T 2 -weighted imaging (T 2 WI), T 1 map, and T 2 map of SSM with different SiO 2 thickness and in different pH environment (incubated 24 h) were measured on a 3.0 T MRI scanner (GE signa HDx, USA). The acquisition parameters were set as: T 1 WI, repetition time (TR) = 500 ms, echo time (TE) = 12 ms, slice thickness = 1 mm, slice spacing = 1 mm, FOV = 10 × 10 cm, matrix = 256 × 256; T 1 Map images, TR = 4.0 ms, TE = 2.0 ms, slice thickness = 1 mm, slice spacing = 1 mm, FOV = 10 × 10 cm, matrix = 256 × 256; T 2 WI, TR = 2500 ms, TE = 60 ms, slice thickness = 1 mm, slice spacing = 1 mm, FOV = 10 × 10 cm, matrix = 256 × 256; T 2 Map images, TR = 1000 ms, TE = 12 − 180 ms, slice thickness = 1 mm, slice spacing = 1 mm, FOV = 10 × 10 cm, matrix = 256 × 256. Quantitative T 1 and T 2 relaxation maps were reconstructed from datasets via Paravision 4 software. The same method was applied for the pH sensitivity evaluation of SSM in different pH conditions. In vitro MR imaging To evaluate the pH sensitivity in vitro, We chose different cell lines to simulate the different pH environments. Renal epithelial cells (293T), breast cancer cells (4T1), and glioma cells (U87) were seeded in 6 cm cell culture dishes (1× 10 6 cells per well) and incubated for 12 h, respectively. SSM-PEG (0.1 mg mL −1 ) was added to each well and incubated for 2 h. the cells were washed three times with PBS, and incubate with fresh medium for another 4 h. After incubation, cells were digested and centrifuged for 5 min at 175 × g and resuspended in 1 mL agarose (0.5 wt.%). The T 1 and T 2 -weighted MR images were acquired using a 3.0 T MR system. For T 2 Map images, the MRI parameters were TR = 1000, TE = 12–180 ms, FOV = 10 × 10 cm, matrix = 256 × 256. For T 1 Map images, the MRI parameters were TR = 4.0 ms, TE = 2.0 ms, FOV = 10 × 10 cm, matrix = 256 × 256. The mean T 1 and T 2 relaxation times (ms) were measured for each sample. Quantitative T 1 and T 2 maps were reconstructed from datasets using MATLAB software. To investigate the time dependence properties, 293T cells and 4T1 cells were seeded in 6 cm cell culture dishes (1 × 10 6 cells per well) and incubated for 12 h, respectively. SSM-PEG (0.1 mg mL −1 ) was added to each well and incubated for different times (0.5, 1, 2, 4, 8, and 16 h). 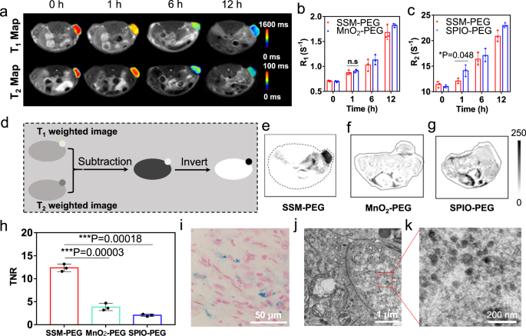Fig. 5: SSM-PEG (PEG-modified SPIO@SiO2@MnO2) for in vivo MRI of 4T1 xenograft tumor-bearing mice. aT1and T2Map,bR1, andcR2at the tumor site of the 4T1-bearing mice. The I.V. injections of SSM-PEG and MnO2-PEG were given a dosage of 5 mg/kg, and the MRI diagnosis was performed at different time points at 0, 1, 6, and 12 h post the injection. T1and T2Map are representative data from three mice samples.R1andR2Data are presented as mean ± SD from three independent mice samples.dIllustration of the Dual-contrast-Enhanced Subtraction Imaging (DESI) procedures; T1and T2dual-modal MRI images were processed by DESI method of the tumor-bearing mice at 12 h after the injection ofeSSM-PEG, f MnO2-PEG, andgSPIO-PEG. Representative data are shown from three mice samples.hThe tumor-to-normal tissue signal ratios (TNRs) quantified from the DESI processed images ine–g. Data are presented as mean ± SD from three independent mice samples.iPrussian blue stain and (j) and (k) TEM images of the tumor slices from the mice receiving the injection of SSM-PEG. Representative data are shown from three mice samples. The two-tailed Student’s t-test is employed for the statistical analysis. *P< 0.05; **P< 0.01; ***P< 0.001. Source data are provided as a Source Data file. And then, the MRI performances were measured according to the method mentioned above. Stability of SPIO@SiO 2 @MnO 2 -PEG (SSM-PEG) The size distribution and zeta potential of SSM before and after PEGylation were observed by dynamic light scattering (DLS) instruments (Malvern, Nano-ZS). The stability of SSM-PEG (0.1 mg mL −1 ) was measured in 10% FBS solution by DLS. Hemolysis test of SPIO@SiO 2 @MnO 2 -PEG (SSM-PEG) The hemolysis of SPIO@SiO 2 @MnO 2 -PEG (SSM-PEG) was investigated using fresh blood from healthy mice (female BALB/c mice, aged 6–8 weeks). The red blood cells (RBCs) were collected by centrifugation at 175 × g for 10 min, washed three times with PBS, and then brought to a final concentration of 2% (v/v) in PBS. Two hundred milliliters of erythrocyte suspension was mixed with different concentrations (0.05 and 0.10 mg mL −1 ) of SSM and SSM-PEG, respectively, and incubated for 4 h at 37 °C in an incubator shaker. The mixtures were centrifuged at 175 × g for 5 min, and the supernatants (100 μL) of all samples were transferred to a 96-well plate. Free hemoglobin in the supernatant was measured by the absorbance at 540 nm using a microplate reader (Cytation 3 microplate reader, BioTek Instruments, Inc., Winooski, USA). RBC incubated with DI water and PBS buffer were used as the positive and negative controls, respectively. Cytotoxicity To evaluate the cytotoxicity of SSM before and after PEGylation, 4T1 cells seeded in 96-well plates were pre-incubated with different concentrations of SSM and SSM-PEG (normalized by the concentration of iron: 0.2, 0.4, 2.0, 4.0, 20, 40 μM). After a 24-h incubation, the cells were gently washed by PBS buffer three times to remove the non-internalized nanoparticles. The cell viabilities were determined by MTT assay, and the results were presented as average ± SD ( n = 3). Pharmacokinetic analyses The pharmacokinetics of SSM and SSM-PEG were systematically investigated using Inductively Coupled Plasma Mass Spectrometry (ICP-MS, Agilent 7700x) for the quantified amount of Fe in the blood samples. Briefly, the blood samples were collected at different time points (5, 10, 20 30 min, 1, 2, 4, and 24 h) after the administration of SSM and SSM-PEG (10 mg kg −1 ) via intravenous injection (female BALB/c mice, aged 6–8 weeks, 3 mice per group). In vivo MR imaging of subcutaneous xenograft model All animal experiments were in accord with Institutional Animal Use and Care Regulations, approved by the Laboratory Animal Ethics Committee of the Southern University of Science and Technology (No. SUSTC-JY2019068) and Shanghai General Hospital. To establish subcutaneous tumors in mice, 4T1 cells were harvested by centrifugation, washed, and resuspended in PBS (2 × 10 7 cells mL −1 ). A 100-μL cell suspension containing 2 × 10 6 cells was then injected subcutaneously into the right flank of the female BALB/c mice (aged 6–8 weeks, 1 site per mice). When tumors were well established and had reached diameters of 6–8 mm (tumors were measured with vernier caliper, and the volume was calculated by V = 0.5 × length × width 2 ; for both single and bilateral flank tumor models, mice were sacrificed when the total tumor burden exceeded 2000 mm 3 ), the mice were used for in vivo MR imaging. Mice bearing with 4T1 breast tumor were scanned on a 3.0 T MR system with a high-resolution animal coil at 0, 1, 6, and 12 h after tail vein injection of the SPIO-PEG, MnO 2 -PEG, and SSM-PEG (100 μL each, normalized by SPIO concentration of 1 mg mL −1 , SPIO-PEG was set as the T 2 control group, and MnO 2 -PEG was set as the T 1 control group, n = 3). All mice were imaged under the T2WI spin-echo sequence (TR/TE 2000/60 ms) and T 1 WI spin-echo sequence (TR/TE 450/12 ms) with a 256 × 256 matrix size. The mean T 2 -weighted signal intensities and T 1 -weighted signal intensities were measured for each tumor. For T 2 Map images (TR = 1000, TE = 12–180 ms, FOV = 12 × 12 cm, matrix = 256 × 256) and T 1 Map images (TR = 4.0 ms, TE = 2.0 ms, FOV = 12 × 12 cm, matrix = 256 × 256) were obtained with a 3.0 T MRI. The mean T 2 relaxation time and T 1 relaxation time were measured for each tumor. Quantitative T 2 maps and T 1 maps were reconstructed from datasets using MATLAB software. In vivo MR imaging of liver metastatic models To prepare the liver metastatic models, the spleen was exposed through the incision, 4T1 cells (1 × 10 5 ) were suspended in 50 μL PBS and injected into the edge of the spleen (female nude mice at the age of 6–8 weeks), then the mouse was sutured. 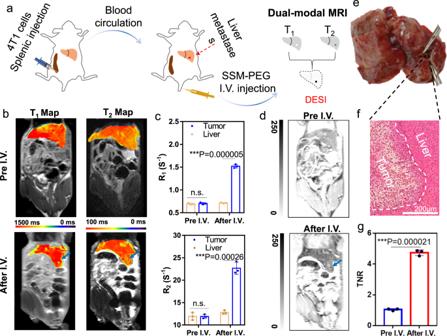Fig. 6: SSM-PEG (PEG-modified SPIO@SiO2@MnO2) for MRI trace of tiny liver metastases in vivo. aIllustration of the construction and MRI diagnosis processes of the metastatic model.bT1and T2map images andcR1andR2at the liver metastasis of the mice before I.V. injection and 2 h after the injection of SSM-PEG. T1and T2Map are representative data from three mice samples. R1and R2Data are presented as mean ± SD from three independent mice samples.dT1and T2dual-modal MRI images of the liver metastasis were processed by DESI method, which were taken without the use of contrast agent and 2 h after the injection of SSM-PEG. Representative data are shown from three mice samples.eEx vivo image of the liver with a tiny metastasis. Representative data are shown from three mice samples.fH&E stain of the slices of the liver metastasis. Representative data are shown from three mice samples.gTNR quantified from the DESI processed images in d and e. Data are presented as mean ± SD from three independent mice samples. The two-tailed Student’st-test is employed for the statistical analysis. *P< 0.05; **P< 0.01; ***P< 0.001. Source data are provided as a Source Data file. 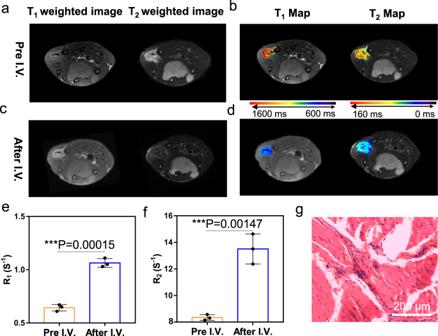Fig. 7: SSM-PEG (PEG-modified SPIO@SiO2@MnO2) for MRI diagnosis of inflammation in vivo. aT1and T2weighted images andbT1& T2Map of muscle inflammation without the use of contrast agents. Representative data are shown from three mice samples.cT1and T2weighted images anddT1and T2Map of muscle inflammation of the rats receiving I.V. injection of SSM-PEG. Representative data are shown from three mice samples.eR2andfR1at the muscle inflammation sites before and after 2 h injection of SSM-PEG contrast agents. Data are presented as mean ± SD from three independent mice samples.gH&E stain of tissue slices taken from the muscle inflammation sites. Representative data are shown from three mice samples. The two-tailed Student’st-test is employed for the statistical analysis. *P< 0.05; **P< 0.01; ***P< 0.001. Source data are provided as a Source Data file. Two weeks later, these mice were collected for in vivo MR imaging. Mice bearing with 4T1 breast tumor were scanned on a 3.0 T MR system with a high-resolution animal coil at 0 h and 2 h after tail vein injection of the SSM-PEG (100 μL, by SPIO concentration of 1 mg mL −1 , n = 3). All mice were imaged under the T 2 WI spin-echo sequence (TR/TE 2000/60 ms) and T 1 WI spin-echo sequence (TR/TE 450/12 ms) with a 256 × 256 matrix size. The mean T 2 -weighted signal intensities and T 1 -weighted signal intensities were measured for each tumor (Smean). For T 2 Map images (TR = 1000, TE = 12–180 ms, FOV = 12 × 12 cm, matrix = 256 × 256) and T 1 Map images (TR = 4.0 ms, TE = 2.0 ms, FOV = 12 × 12 cm, matrix = 256 × 256) were obtained with a 3.0 T MRI. The mean T 2 relaxation time and T 1 relaxation time were measured for each tumor. Quantitative T 2 Maps and T 1 Maps were reconstructed from datasets using MATLAB software. In vivo MR imaging of inflammation model Female nude rats at 4 weeks of age were obtained from Charles River Laboratory Animal Technology Co., Ltd. (Beijing, China). To establish inflammation model in rats, turpentine (20 μL) was injected into the thigh muscle of rats. After 1 week, SSM-PEG was intravenously injected, and the MRI measurements were performed ( n = 3). All rats were imaged under the T 2 WI spin-echo sequence (TR/TE 2000/60 ms) and T 1 WI spin-echo sequence (TR/TE 450/12 ms) with a 256 × 256 matrix size. The mean T 2 -weighted signal intensities and T 1 -weighted signal intensities were measured for each tumor (Smean). For T 2 Map images (TR = 1000, TE = 12–180 ms, FOV = 12 × 12 cm, matrix = 256 × 256) and T 1 Map images (TR = 4.0 ms, TE = 2.0 ms, FOV = 12 × 12 cm, matrix = 256 × 256) were obtained with a 3.0T MRI. The mean T 2 relaxation time and T 1 relaxation time were measured for each tumor. Quantitative T 2 Maps and T 1 Maps were reconstructed from datasets using MATLAB software. H&E staining and Prussian blue staining After humanely killing the mice, we collected the major organs and tumors, which were fixed in 4% paraformaldehyde. The organs were then sliced and stained by H&E (Hematoxylin-Eosin staining) to evaluate the systemic toxicity of the contrast agents. The tumor was also sliced and stained by Prussian Blue, which was performed to detect iron uptake in cells. Blood routine tests The blood of healthy mice and the tumor-bear mice with the injection of SSM-PEG were collected and proceeded to blood routine tests on an automatic hematology analyzer (DF52Vet, Dymind Biotech., China). Statistics and reproducibility All of the experimental data were obtained in triplicate unless otherwise mentioned and are presented as mean ± SD. Statistical comparison by analysis of variance was performed at a significance level of P < 0.05 based on a Student’s t -test. Reporting summary Further information on research design is available in the Nature Portfolio Reporting Summary linked to this article.